BCLAF1 and its splicing regulator SRSF10 regulate the tumorigenic potential of colon cancer cells Bcl-2-associated transcription factor 1 (BCLAF1) is known to be involved in multiple biological processes. Although several splice variants of BCLAF1 have been identified, little is known about how BCLAF1 splicing is regulated or the contribution of alternative splicing to its developmental functions. Here we find that inclusion of alternative exon5a was significantly increased in colorectal cancer (CRC) samples. Knockdown of the BCLAF1 protein isoform resulting from exon5a inclusion inhibited growth and that its overexpression increased tumorigenic potential. We also found that the splicing factor SRSF10 stimulates inclusion of exon5a and has growth-inducing activity. Importantly, the upregulation of SRSF10 expression observed in clinical CRC samples parallels the increased inclusion of BCLAF1 exon5a, both of which are associated with higher tumour grade. These findings identify SRSF10 as a key regulator of BCLAF1 pre-mRNA splicing and the maintenance of oncogenic features in human colon cancer cells. Bcl-2-associated transcription factor 1 (BCLAF1) has been reported to be involved in diverse biological processes. It was initially identified as a protein partner for the adenoviral bcl-2 homologue E1B19K. Forced expression of BCLAF1 can induce apoptosis in HeLa cells [1] , suggesting a role for BCLAF1 in apoptotic signalling. However, the role in apoptotic pathway remains controversial, as cells from BCLAF1-deficient mice do not have obvious defects in apoptosis [2] . Indeed, multiple functions have been described for BCLAF1 by different groups, such as in posttranscriptional processes [3] , [4] , production of Kaposi's sarcoma-associated herpesvirus [5] and human cytomegalovirus infection [6] , lung development and T-cell activation [2] , [7] . Multiple transcript variants encoding different isoforms that are generated by alternative splicing have been found for BCLAF1 gene, and perhaps the functional discrepancies among BCLAF1-related studies reflect the possible specificity for different protein isoform in certain cellular contexts. Alternative splicing is a regulated process that involves various cis -acting RNA elements (enhancers or silencers) bound by different splicing regulators, which may act synergistically or antagonistically to determine whether an alternative exon is included or excluded [8] , [9] , [10] . In fact, majority of multi-exon human genes undergo alternative splicing to produce tissue- or developmental stage-specific splice variants [11] , [12] , and more than half of them can be subsequently translated into diverse protein isoforms with distinct functions [13] . However, it remains to be defined how splicing factors regulate alterative splicing of BCLAF1 pre-mRNA in various biological processes. Aberrant alternative splicing events are commonly observed in cancer cells and have been implicated in many types of cancer [14] , [15] . For example, many genes that are involved in proliferation and invasiveness are frequently alternatively spliced, and their specific splice variants, which stimulate cell proliferation and migration, and thus contribute to the transformed phenotype, are often upregulated in tumours. These changes often involve dysregulated expression of RNA-binding proteins [16] and/or protein kinases that regulate their activities [17] , [18] . SR proteins (Serine/arginine-rich proteins) are well-characterized RNA-binding proteins that play critical roles in splicing regulation, and changes in the expression of these proteins can dramatically affect alternative splicing profiles in cells [8] , [9] , [10] . However, the roles of spliced variants and splicing factors that control splicing misregualtion are not completely appreciated in tumour development. In this study, we observed that inclusion of BCLAF1 exon5a was significantly increased in colon cancer cell lines and colorectal cancer (CRC) samples. 5a-containing and -lacking BCLAF1 transcripts produce two protein isoforms—full-length isoform (L isoform) and truncated isoform (T isoform)—with L isoform prevalent in colon cancer cell lines. Isoform-specific knockdown of BCLAF1-L inhibits cell growth and colony formation in vitro , and significantly decreased tumour formation in nude mice. Overexpression of BCLAF1-L considerably increased colony-forming efficiency of cells, suggesting pro-tumorigenic capacity for the L isoform in colon cancer cells. Mechanism analysis demonstrated that splicing factor SRSF10 (serine/arginine-rich splicing factor 10), an atypical member of SR proteins and a key regulator of alterative splicing in vivo [19] , [20] , [21] , specifically binds to exon5a. SRSF10 activates the inclusion of exon5a, as its loss leads to a dramatic shift of exon5a-containing product to exon5a-lacking product in colon cancer cells. We further demonstrated that SRSF10 knockdown also dramatically inhibited growth of colon cancer cells, colony formation in vitro and tumorigenesis in vivo , which are comparable to the effects observed on BCLAF1-L knockdown in these cells and in a mouse xenograft model. Specific splice-switching oligonucleotides (SSO) targeted against BCLAF1 exon5a and introduction of BCLAF1-L isoform into SRSF10 knockdown cells further demonstrated that SRSF10 regulation of BCLAF1 pre-mRNA splicing plays an important role in mediating tumorigenesis of colon cancer cells. Importantly, upregulation of SRSF10 that was observed in clinical CRC samples remarkably parallels the increased BCLAF1 exon5a inclusion, both of which are closely related with the higher tumour grade. Therefore, our study strongly highlights the biological significance of the BCLAF1-L isoform and SRSF10 in the colorectal tumorigenesis and identifies SRSF10 as a key regulator for controlling BCLAF1 pre-mRNA splicing and thus maintaining oncogenic phenotypes of colon cancer cells. Disregulated BCLAF1 exon5a splicing in clinical CRC samples Human BCLAF1 has 13 exons; both exon5a and exon11 are subject to alternative splicing regulation, which generates four different transcript variants dependent on inclusion/exclusion of these regulated exons ( Fig. 1a , top). Interestingly, high sequence similarity is observed over the entire coding region of BCLAF1 among 46 vertebrates examined, especially over the exon4 and exon5a, while their flanking intronic sequences are much less conserved. Specifically, it shares 96% and 91% amino acid identity between mouse to human and between chicken to human, respectively ( Fig. 1a , bottom). This perhaps indicates vital functions for BCLAF1 in vivo . 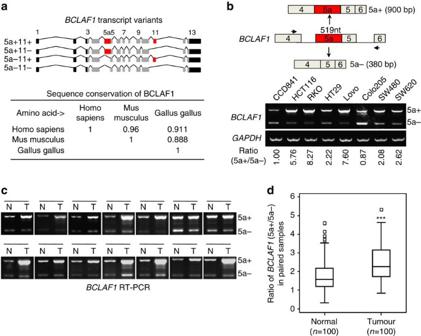Figure 1: Inclusion ofBCLAF1exon5a is increased in CRC samples. (a) Top: schematic diagram ofBCLAF1splice variants. Constitutive exons are shown as grey and black boxes: grey represents coding regions and black for untranslated regions, while red boxes —alternatively spliced coding regions—including exon5a and exon11. (Bottom) Sequence conservation was compared for BCLAF1 among the indicated three species. (b) Top: diagrams for detection ofBCLAF1variants including or lacking alternative exon 5a (5a+ or 5a−). Primer pairs and product sizes for the two variants are shown. Bottom: inclusion of exon5a was examined in one normal colon epithelial cell line (CCD841) and seven cancer cell lines (HCT116, RKO, HT29, Lovo, Colo205, SW480 and SW620) by RT–PCR. Ratio for 5a+/5a− is listed below the panel. (c) Total RNAs from 100 paired human CRC and normal tissues were examined by RT–PCR using primer sets described inb. Representative results for detection ofBCLAF1exon5a splicing patterns are shown between CRC (T) and matched normal tissues (N) from the same patient. (d) Quantification of data fromcfor exon5a inclusion/exclusion ratio. Three PCRs were quantified and averaged for each sample. The median box and whiskers plot was then calculated for the paired normal and tumour sets using SAS software. Figure 1: Inclusion of BCLAF1 exon5a is increased in CRC samples. ( a ) Top: schematic diagram of BCLAF1 splice variants. Constitutive exons are shown as grey and black boxes: grey represents coding regions and black for untranslated regions, while red boxes —alternatively spliced coding regions—including exon5a and exon11. (Bottom) Sequence conservation was compared for BCLAF1 among the indicated three species. ( b ) Top: diagrams for detection of BCLAF1 variants including or lacking alternative exon 5a (5a+ or 5a−). Primer pairs and product sizes for the two variants are shown. Bottom: inclusion of exon5a was examined in one normal colon epithelial cell line (CCD841) and seven cancer cell lines (HCT116, RKO, HT29, Lovo, Colo205, SW480 and SW620) by RT–PCR. Ratio for 5a+/5a− is listed below the panel. ( c ) Total RNAs from 100 paired human CRC and normal tissues were examined by RT–PCR using primer sets described in b . Representative results for detection of BCLAF1 exon5a splicing patterns are shown between CRC (T) and matched normal tissues (N) from the same patient. ( d ) Quantification of data from c for exon5a inclusion/exclusion ratio. Three PCRs were quantified and averaged for each sample. The median box and whiskers plot was then calculated for the paired normal and tumour sets using SAS software. Full size image We first investigated expression levels of BCLAF1 splice variants in various mouse tissues. To this end, we designed primer pairs that detect alternative exon5a and 11, respectively ( Fig. 1b ). Reverse transcription–PCR (RT–PCR) revealed that inclusion of exon5a appears tissue-specific, while exon11 is included more frequently in all the tissues examined ( Supplementary Fig. 1 ). For example, the 5a-containting (5a+) transcript is more prevalent in the heart, liver, spleen and testis, but less frequently used in the skeletal muscles and stomach. We next examined splicing patterns of BCLAF1 pre-mRNA in different human cancer cell lines. Although inclusion of exon11 remains largely the same in all the cancer and normal cell lines examined ( Supplementary Fig. 2 ), the ratio for inclusion versus exclusion of exon5a was significantly elevated in six of seven colon cancer cell lines, compared with that obtained from normal colon epithelial cells ( Fig. 1b ). However, this increase was not significantly observed between normal cell lines and lung and breast cancer cell lines ( Supplementary Fig. 2 ). As inclusion of exon11 is very common in mouse tissues and different cancer cell lines, inclusion or exclusion of exon5a would make a major contribution to the generation of protein isoforms. Translation of the exon5a-included mRNA gives a large protein of 920 amino acids (L isoform, see below), while the exon5a-lacking transcript generates a truncated protein of 747 amino acids (T isoform, see below). Our data reveal that BCLAF1-L is the major isoform of BCLAF1 in colon cancer cells and suggest that the L isoform might play a role in colorectal tumorigenesis. We next compared the ratio of BCLAF1 5a+/5a− mRNA in clinical CRC samples. One hundred human CRC tissues paired with their adjacent non-cancerous tissues were examined. Representative RT–PCR results are shown in Fig. 1c and quantification of BCLAF1 splice variants from three independent experiments as in Fig. 1d . We observed consistent levels of exon5a inclusion versus exclusion in normal tissues (1.79±0.81, n =100), whereas inclusion of exon5a in tumour samples was increased by a mean value of 35% (2.42±0.95, n =100) ( Fig. 1d ). Approximately a 1.5-fold increase between exon5a+/5a− (T) and exon5a+/5a− (N) was observed in 45% of the cancer samples compared with non-cancerous colorectal tissues ( Table 1 ). Importantly, increased exon5a inclusion is probably associated with the higher tumour grade ( P =0.0056; Table 1 ). These data suggest that the L isoform plays a role in the development of CRC. Table 1 Relationship between ratios of BCLAF1 exon5a+/exon5a− in colorectal carcinoma and clinical and pathological features of the individuals. Full size table Oncogenic role of BCLAF1-L in human colon cancer cells To test whether BCLAF1-L promotes cell proliferation, we designed two different small interfering RNAs (siRNAs) targeted against exon5a for isoform-specific knockdown of BCLAF1-L. As shown in Fig. 2a , a prominent band of ~140 kDa (L isoform) and another minor product of 110 kDa (T isoform) were readily detected in RKO cells (lane 1). Treatment with specific L1 or L2 siRNA significantly decreased levels of the L isoform, but has no effects on the expression of T isoform, compared with control siRNA ( Fig. 2a ). 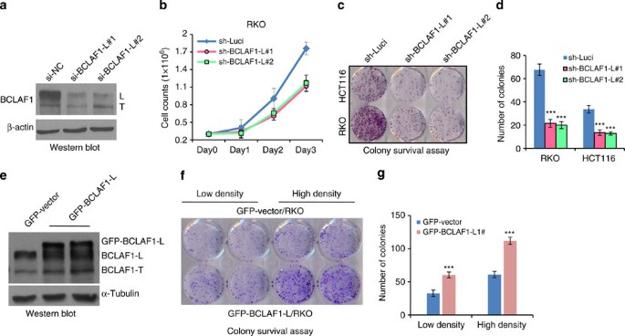Figure 2: BCLAF1-L is required for survival of colon cancer cells. (a) RKO cells were treated for 72 h with the indicated siRNAs. BCLAF1-L knockdown was assessed by western blotting using β-actin as a loading control. (b) Cell proliferation assay. RKO cells were infected with retroviruses expressing shRNA-BCLAF1-L1, L2 or control shRNA, and selected for puromycin resistance. Cell proliferation was measured by trypan blue exclusion. (c,d) Clonogenic survival assay and quantification of RKO and HCT116 cells either stably expressing shLuci or each of shRNA-L1 and L2 as described inb. Three independent experiments were performed and representative cells stained with crystal violet were shown. The number of focal adhesions was quantified in the right bar graph and results are shown as mean±s.d. (e) RKO cells were transfected with GFP-BCLAF1-L plasmid and selected for neomyocin resistance. Overexpression of BCLAF1-L was confirmed by western blotting. (f,g) Clonogenic survival assay and quantification was performed with RKO cells stably expressing GFP-BCLAF1-L as described inc,d. All experiments were repeated three times and results are shown as mean±s.d. Figure 2: BCLAF1-L is required for survival of colon cancer cells. ( a ) RKO cells were treated for 72 h with the indicated siRNAs. BCLAF1-L knockdown was assessed by western blotting using β-actin as a loading control. ( b ) Cell proliferation assay. RKO cells were infected with retroviruses expressing shRNA-BCLAF1-L1, L2 or control shRNA, and selected for puromycin resistance. Cell proliferation was measured by trypan blue exclusion. ( c , d ) Clonogenic survival assay and quantification of RKO and HCT116 cells either stably expressing shLuci or each of shRNA-L1 and L2 as described in b . Three independent experiments were performed and representative cells stained with crystal violet were shown. The number of focal adhesions was quantified in the right bar graph and results are shown as mean±s.d. ( e ) RKO cells were transfected with GFP-BCLAF1-L plasmid and selected for neomyocin resistance. Overexpression of BCLAF1-L was confirmed by western blotting. ( f , g ) Clonogenic survival assay and quantification was performed with RKO cells stably expressing GFP-BCLAF1-L as described in c , d . All experiments were repeated three times and results are shown as mean±s.d. Full size image Given the role ascribed to BCLAF1 in apoptosis [1] , we sought to determine whether BCLAF1-L knockdown affects the cellular response to apoptotic stimuli. However, no difference in cell death induction was observed in control cells and BCLAF1-L knockdown cells following treatment with five different apoptosis inducers ( Supplementary Fig. 3 ). Next, we assessed the effects of BCLAF1-L depletion on cell proliferation. As shown in Fig. 2b , stable expression of BCLAF1-L1 or 2 short hairpin RNA (shRNA) reduced growth rate of RKO cells in comparison with control cells expressing Luci (Luciferase) shRNA. We then checked effects of BCLAF1-L knockdown on clonogenic survival of colon cancer cells. Strikingly, BCLAF1-L knockdown considerably reduced colony formation of both RKO and HCT116 cells ( Fig. 2c,d ). These findings suggest that BCLAF1-L appears to be dispensable for execution of cell death pathways but is required for cancer cell growth and survival. To further corroborate this hypothesis, we tested whether overexpression of BCLAF1-L might promote colony formation of colon cancer cells. To this end, we generated RKO cell pools stably expressing green fluorescent protein (GFP)-tagged BCLAF1-L ( Fig. 2e ). In accordance with effects of BCLAF1 knockdown, overexpression of the L isoform significantly increased colony-forming efficiency of RKO cells ( Fig. 2f,g ), further confirming its pro-tumorigenic function in colon cancer cells. BCLAF1-L isoform promotes tumorigenesis of RKO cells in mice To explore underlying mechanisms of pro-tumorigenic effects of the L isoform, microarray analysis was performed using total RNA prepared from RKO/shBCLAF1-L1 and control cells. Gene Ontology analysis revealed that BCLAF1-L knockdown specifically decreased expression of genes involved in the regulation of intercellular adhesion and cytockeletal architecture ( Fig. 3a and Supplementary Table 1 ). RT–PCR further validated differentially expressed genes in both BCLAF1-L knockdown cell lines. As shown in Fig. 3b , four of the most downregulated genes affect mediators of cytoskeletal organization ( ENAH , MSN ) or extracellular matrix proteins ( FN1 , ITGA1 ). Overexpression of these genes has been observed in different human cancers, including CRCs [22] , [23] , [24] , [25] . Interestingly, three of them were upregulated at mRNA levels in cells overexpressing the L isoform ( Supplementary Fig. 4a ), suggesting their important roles in the L isoform-mediated effects in colon cancer cells. Among the upregulated genes, a more than twofold increase was observed in the expression of tumour suppressor genes such as Spry2 (ref. 26 ), AKAP12 (ref. 27 ) and RASSF8 (ref. 28 ), which are often downregulated in human colon cancers. However, for the known targets reported for BCLAF1, such as CCND1 and TP53 , there were no significant changes observed after BCLAF1-L knockdown ( Supplementary Fig. 4b ). 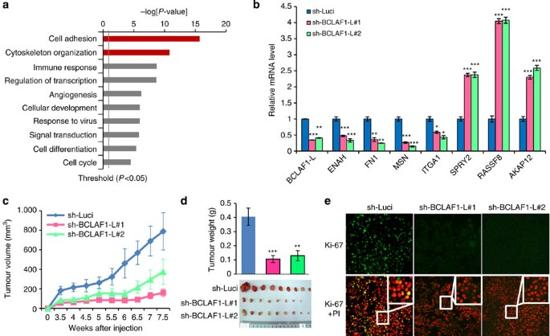Figure 3: BCLAF1-L knockdown inhibits xenograft growth of RKO cells. (a) Top significant biological processes for genes differentially expressed in BCLAF1-L-depleted RKO cells. Cell adhesion and cytoskeleton organization are the most affected biofunction affected by BCLAF1-L knockdown. (b) Validation of microarray results by real-time PCR on eight genes predicted from the microarray analysis was performed. The experiments were repeated at least three times, and results are shown as mean±s.d. (c) Time-course of xenograft growth. Stable RKO/sh-BCLAF1-L1, RKO/sh-BCLAF1-L2 and RKO/sh-Luci cells described inFig. 2bwere injected into nude mice, and tumour volumes were measured every half of week. Each point represents the mean volume±s.d. of tumours. (d) Tumour weight. Mice described incwere killed at 7.5 weeks after injection. Tumours were excised from the mice and weighted. Results are shown as mean±s.d. of tumour weights (n=9, 8, 9 per group, respectively, each with initial 12 injections). (e) Tumours shown indwere formalin-fixed, paraffin-embedded and sliced for Ki-67 staining. Ki-67 (green signal) stains the nucleus region of proliferating cells and propidium iodide (PI, red signal) stains for nuclei of all cells; hence, the merged yellow signal indicates proliferating cells. Figure 3: BCLAF1-L knockdown inhibits xenograft growth of RKO cells. ( a ) Top significant biological processes for genes differentially expressed in BCLAF1-L-depleted RKO cells. Cell adhesion and cytoskeleton organization are the most affected biofunction affected by BCLAF1-L knockdown. ( b ) Validation of microarray results by real-time PCR on eight genes predicted from the microarray analysis was performed. The experiments were repeated at least three times, and results are shown as mean±s.d. ( c ) Time-course of xenograft growth. Stable RKO/sh-BCLAF1-L1, RKO/sh-BCLAF1-L2 and RKO/sh-Luci cells described in Fig. 2b were injected into nude mice, and tumour volumes were measured every half of week. Each point represents the mean volume±s.d. of tumours. ( d ) Tumour weight. Mice described in c were killed at 7.5 weeks after injection. Tumours were excised from the mice and weighted. Results are shown as mean±s.d. of tumour weights ( n =9, 8, 9 per group, respectively, each with initial 12 injections). ( e ) Tumours shown in d were formalin-fixed, paraffin-embedded and sliced for Ki-67 staining. Ki-67 (green signal) stains the nucleus region of proliferating cells and propidium iodide (PI, red signal) stains for nuclei of all cells; hence, the merged yellow signal indicates proliferating cells. Full size image We next examined the role of BCLAF1-L in tumorigenesis in vivo . RKO cells stably expressing L1 or L2 shRNA were injected into the flanks of 4-week-old nude mice (see Methods). Knockdown of BCLAF1-L decreased the tumour growth rate and tumour size ( Fig. 3c,d ), indicating that BCLAF1-L stimulates in vivo tumour growth. To disclose the underlying mechanisms responsible for the decreased tumorigenesis, we examined the influence of BCLAF1-L knockdown on cell proliferation and apoptosis in vivo . Although BCLAF1-L knockdown had no significant effect on cell apoptosis, as demonstrated by TUNEL (TdT-mediated dUTP nick end labelling) assay ( Supplementary Fig. 5 ), Ki67 staining of xenografts derived from RKO/sh-BCLAF1-L1 and 2 cells indicated that cell proliferation was dramatically decreased ( Fig. 3e ), which was consistent with our in vitro observation. These results indicate that the tumour-stimulating effect of BCLAF1-L is mainly attributed to its role in facilitation of tumour cell growth. BCLAF1 is a conserved transcript target regulated by SRSF10 The mechanism controlling exon5a inclusion is currently unknown. To identify regulatory cis -elements that modulate exon5a splicing and the corresponding trans -acting factors, we first examined the sequence of exon5a for the presence of potential binding sites for RNA-binding proteins. Strikingly, we found many purine-rich (GA rich) motifs especially within the downstream 200 bp region (5a3) of exon5a, and each constitutes a good match to the binding motif of splicing factor SRSF10 (previously known as SRp38; Supplementary Fig. 6a ) [21] , [29] . Neither exon5 nor exon11 contained a match to the SRSF10 consensus sequence. SRSF10 is an atypical SR protein that functions as a sequence-dependent splicing activator as well as a key regulator of alternative splicing [19] , [20] , [21] . Motif analysis of SRSF10-regulated splicing events in vivo revealed that the binding of SRSF10 to the alternative exon is associated with exon inclusion [21] . To determine whether SRSF10 specifically binds exon5a to activate its inclusion, we prepared 32 P-labelled 5a1, 5a2 and 5a3 RNA, each containing the putative SRSF10 binding sites, and compared binding in gel shift assays with exon5 RNA. The results indicate that SRS10 preferably binds to 5a1, 5a2 and 5a3 RNAs as compared with its weak binding to the constitutive exon5 RNA ( Fig. 4a ). To further measure whether SRSF10 binds exon5a mRNA in vivo , we transiently overexpressed haemagglutinin (HA)-tagged SRSF10 complementary DNA in 293T cells ( Fig. 4b ). After ultraviolet irradiating the cells, we isolated cross-linked adducts by immunoprecipitation with immobilized anti-HA-tag antibody. We then purified the bound mRNA and analysed it by RT–PCR, using primers specific for either exon5a1, 5a2 and 5a3, or exon5. Consistent with the above gel-shift results, SRSF10 specifically bound to 5a1, 5a2 and 5a3 RNA, compared with empty-vector control ( Fig. 4c , compare lane 6 and lane 5). In addition, two other SR proteins, SRSF1 and SRSF2, did not display significant affinity for exon5a RNA compared with exon5 RNA ( Fig. 4c , compare lanes 7–8 and lane 6). 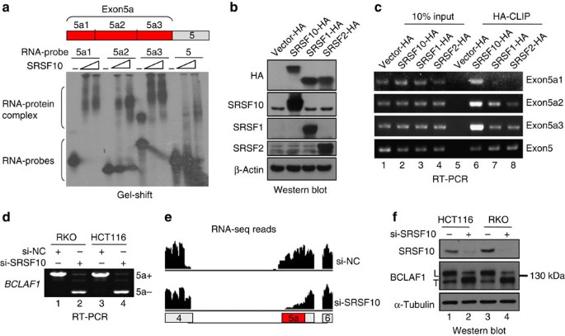Figure 4:BCLAF1was a conserved and direct target of SRSF10. (a) Diagram of exon5a (5a1, 5a2 and 5a3) and exon5 RNA, and gel-shift assays. Indicated32P-labelled RNAs were incubated with increasing amounts of recombinant His-SRSF10 (100 and 300 ng) and complexes were resolved by non-denaturing PAGE. (b) 293T cells were transiently transfected with HA-tagged SRSF10, SRSF1, SRSF2 or empty-vector controls. Western blotting analysis was performed to confirm the expression of each protein by using indicated antibodies. (c)In vivoultraviolet cross-linking and immunoprecipitation (CLIP) from 293T cells described inbwith primer pairs complementary to humanBCLAF1exon5a1, 5a2 and 5a3 or exon5 by RT–PCR. (d) RNAs were extracted from SRSF10 siRNA (si-SRSF10)- and control siRNA (si-NC) -transfected cells. RT–PCR was performed as described inFig. 1b. (e) Schematic diagram of RNA-seq reads coverage overBCLAF1exons 4–6 between si-NC and si-SRSF10 cells. (f) Whole-cell lysates were prepared from cells described indand analysed by western blotting using indicated antibodies. Figure 4: BCLAF1 was a conserved and direct target of SRSF10. ( a ) Diagram of exon5a (5a1, 5a2 and 5a3) and exon5 RNA, and gel-shift assays. Indicated 32 P-labelled RNAs were incubated with increasing amounts of recombinant His-SRSF10 (100 and 300 ng) and complexes were resolved by non-denaturing PAGE. ( b ) 293T cells were transiently transfected with HA-tagged SRSF10, SRSF1, SRSF2 or empty-vector controls. Western blotting analysis was performed to confirm the expression of each protein by using indicated antibodies. ( c ) In vivo ultraviolet cross-linking and immunoprecipitation (CLIP) from 293T cells described in b with primer pairs complementary to human BCLAF1 exon5a1, 5a2 and 5a3 or exon5 by RT–PCR. ( d ) RNAs were extracted from SRSF10 siRNA (si-SRSF10)- and control siRNA (si-NC) -transfected cells. RT–PCR was performed as described in Fig. 1b . ( e ) Schematic diagram of RNA-seq reads coverage over BCLAF1 exons 4–6 between si-NC and si-SRSF10 cells. ( f ) Whole-cell lysates were prepared from cells described in d and analysed by western blotting using indicated antibodies. Full size image We next asked whether SRSF10 could activate splicing of exon5a in vivo . To this end, we used siRNA targeting SRSF10 mRNA and examined the effects of SRSF10 depletion on inclusion of exon5a in RKO and HCT116 cell lines by RT–PCR ( Fig. 4d ). Western blotting confirmed that siRNA-mediated transient elimination of SRSF10 (si-SRSF10) was very efficient in both cells ( Fig. 4f ). Strikingly, inclusion of BCLAF1 exon5a was almost completely skipped on SRSF10 knockdown ( Fig. 4d , compare lanes 2, 4 with lanes 1, 3). Fully in line with this observation, RNA-seq analysis of SRSF10 knockdown RKO cells further confirmed that inclusion of exon5a was directly regulated by SRSF10 ( Fig. 4e ). As BCLAF1 is a highly conserved gene between human and chicken, changes of exon 5a were also observed in chicken cell lines depleted of SRSF10 (ref. 30 ) ( Supplementary Fig. 6b ). We next asked whether the relative expression level of BCLAF1 protein isoforms could be changed by SRSF10 depletion, as judged by western blotting. Consistent with the observed shifts in BCLAF1 5a+/5a− mRNA variants ( Fig. 4d ), SRSF10 knockdown caused a dramatic L–T isoform switch in both human colon cancer cells and chicken cells ( Fig. 4f , compare lane 2 with lane 1, lane 4 with lane 3, and Supplementary Fig. 6c ). Importantly, stable expression of exogenous SRSF10 considerably restored the normal splicing pattern of BCLAF1 in chicken cells both at mRNA and protein levels ( Supplementary Fig. 6b,c ). In addition, knockdown of either SRSF1 or SRSF2 showed on effects on exon5a inclusion ( Supplementary Fig. 7 ). Together, these findings demonstrated that inclusion of exon5a by SRSF10 is consistent with activation mechanism for the protein in splicing regulation [19] , [21] , and strongly indicated that BCLAF1 is a direct splicing target regulated by SRSF10. SRSF10 promotes tumorigenesis via regulating BCLAF1-L levels As SRSF10 is involved in the inclusion of exon5a and thus in the production of BCLAF1-L isoform, we next assessed the effects of SRSF10 depletion on cell proliferation and colony formation in colon cancer cells. Comparable to the effects of BCLAF1-L knockdown, stable expression of SRSF10 shRNA significantly inhibited colon cancer cell growth ( Fig. 5a ) and strongly reduced colony formation in vitro ( Fig. 5b,c ), indicating that BCLAF1 is a major splicing target that mediates the role of SRSF10 in tumour cell growth and survival. These results reflect the loss of SRSF10 rather than an unrelated property of the cells, as a second siRNA against SRSF10 with comparable gene silencing efficacy induced similar effects as the first ( Supplementary Fig. 8 ). 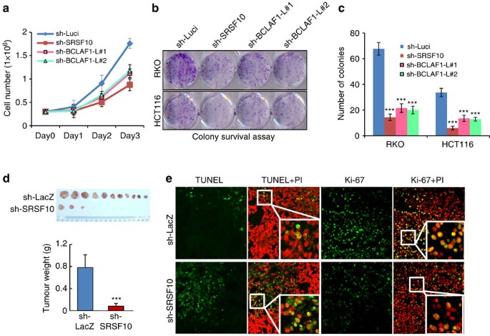Figure 5: SRSF10 is required for tumorigenesis of colon cancer cells. (a) RKO cells were infected with sh-SRSF10 retrovirus and selected for puromyocin resistance. Cell proliferation assay was performed with RKO cells stably expressing sh-SRSF10 along with RKO cells stably expressing sh-BCLAF1-L (1 and 2) for comparison, as described inFig. 2b. (b,c) Clonogenic survival assays and qualification of RKO or HCT116 cells stably expressing sh-SRSF10 or sh-Luci were performed, as described inFig. 2c,d. For comparison, cells stably expressing sh-BCLAF1-L (1 or 2) were also included. Three independent experiments were performed and results are shown as mean±s.d. (d) RKO cells were infected with control or shSRSF10 adenovirus. Twelve hours post infection, the cells were transplanted to nude mice, as described inFig. 3c. After 7 weeks, all the tumours derived from RKO/shSRSF10 or RKO/shLuci cells were shown (top) and tumour weight was measured (bottom), as described inFig. 3d. Results are shown as mean±s.d. of tumour weights (n=11 and 3, respectively, both with initial 12 injections). (e) Tumours shown indwere formalin-fixed, paraffin-embedded and sliced for Ki67 staining and TUNEL assay, as described inFig. 3e. Figure 5: SRSF10 is required for tumorigenesis of colon cancer cells. ( a ) RKO cells were infected with sh-SRSF10 retrovirus and selected for puromyocin resistance. Cell proliferation assay was performed with RKO cells stably expressing sh-SRSF10 along with RKO cells stably expressing sh-BCLAF1-L (1 and 2) for comparison, as described in Fig. 2b . ( b , c ) Clonogenic survival assays and qualification of RKO or HCT116 cells stably expressing sh-SRSF10 or sh-Luci were performed, as described in Fig. 2c,d . For comparison, cells stably expressing sh-BCLAF1-L (1 or 2) were also included. Three independent experiments were performed and results are shown as mean±s.d. ( d ) RKO cells were infected with control or shSRSF10 adenovirus. Twelve hours post infection, the cells were transplanted to nude mice, as described in Fig. 3c . After 7 weeks, all the tumours derived from RKO/shSRSF10 or RKO/shLuci cells were shown (top) and tumour weight was measured (bottom), as described in Fig. 3d . Results are shown as mean±s.d. of tumour weights ( n =11 and 3, respectively, both with initial 12 injections). ( e ) Tumours shown in d were formalin-fixed, paraffin-embedded and sliced for Ki67 staining and TUNEL assay, as described in Fig. 3e . Full size image We next characterized the tumorigenic capacity of SRSF10-depleted cells using human RKO xenograft in nude mice. Figure 5d shows that knockdown of SRSF10 induced a complete loss of tumour formation in 9 of 12 injections. The remaining tumours that formed in RKO/sh-SRSF10 cells demonstrated a dramatic decrease in tumour weight. We then examined the influence of SRSF10 depletion on cell proliferation and apoptosis in vivo . Completely in line with in vitro observations, decreased proliferation was observed in the xenografts derived from RKO/shSRSF10 cells, as demonstrated by Ki67 staining ( Fig. 5e ). Besides, increased apoptosis was also observed in shSRSF10 xenografts ( Fig. 5e ). Overall, these data demonstrate that the loss of SRSF10 dramatically decreases the tumorigenic capacity of colon cancer cells in mice. To provide more evidence that BCLAF1-L mediates the effects of SRSF10 in cancer cell proliferation, we first turned to SSOs (splice-switching oligonucleotides) approach [31] to modulate alternative splicing of BCLAF1 pre-mRNA, which mimics effects of SRSF10 knockdown on the expression of BCLAF1 splice variants ( Fig. 6a ). Compared with control INV-SSO2 treatment, both SSO1 and SSO2 induced increased expression of exon5a-lacking BCLAF1 splice variant ( Fig. 6b ). Consistent with the effects of BCLAF1-L knockdown and SRSF10 knockdown, SSO treatment could strongly reduce cell growth ( Fig. 6c ) and colony-formation capacity of colon cancer cells ( Fig. 6d ). Second, we stably introduced GFP-tagged BCLAF1-L or empty-vector controls into SRSF10 knockdown cells ( Fig. 7a ). Overexpression of the L isoform could significantly increase colony formation in vitro ( Fig. 7b,c ) and tumorigenesis in mice ( Fig. 7d ). In contrast, overexpression of the T isoform has no significant effects observed both in vitro and in vivo ( Fig. 7 ). These data strongly indicate that the reduction in tumorigenesis of SRSF10 knockdown cells is indeed largely due to reduction in the L isoform, further underscoring the importance of SRSF10-mediated splicing regulation of BCLAF1 pre-mRNA in colon cancer cells. 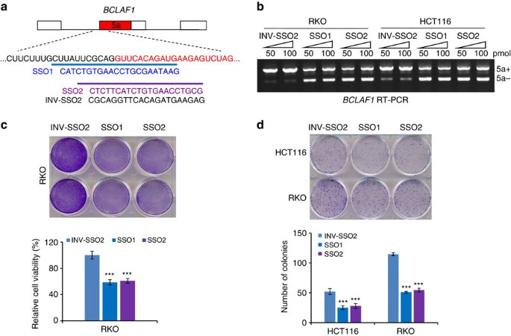Figure 6: Effects of SSOs onBCLAF1alterative splicing modulation. (a) Schematic diagram of splicing-switching oligos SSO1 and SSO2, plus control oligo INV-SSO2 that were designed against 3′-splice site at the boundary of intron4 and exon5a ofBCLAF1pre-mRNA. (b) RKO or HCT116 cells were treated with indicated SSOs. After 96 h, cells were harvested and total RNA was extracted.BCLAF1exon5a splice variants were analysed by RT–PCR. (c) RKO cells were treated with indicated SSO for 72 h and crystal violate staining was performed to show decreased cell viability after SSO treatment. Quantification of relative cell viability was shown below. At least three experiments were repeated and results are shown as mean±s.d. (d) Clonogenic survival assays and qualification of RKO cells after treatment with indicated SSO were performed, as described inFig. 2c,d. The experiments were repeated at least three times and results are shown as mean±s.d. Figure 6: Effects of SSOs on BCLAF1 alterative splicing modulation. ( a ) Schematic diagram of splicing-switching oligos SSO1 and SSO2, plus control oligo INV-SSO2 that were designed against 3′-splice site at the boundary of intron4 and exon5a of BCLAF1 pre-mRNA. ( b ) RKO or HCT116 cells were treated with indicated SSOs. After 96 h, cells were harvested and total RNA was extracted. BCLAF1 exon5a splice variants were analysed by RT–PCR. ( c ) RKO cells were treated with indicated SSO for 72 h and crystal violate staining was performed to show decreased cell viability after SSO treatment. Quantification of relative cell viability was shown below. At least three experiments were repeated and results are shown as mean±s.d. ( d ) Clonogenic survival assays and qualification of RKO cells after treatment with indicated SSO were performed, as described in Fig. 2c,d . The experiments were repeated at least three times and results are shown as mean±s.d. 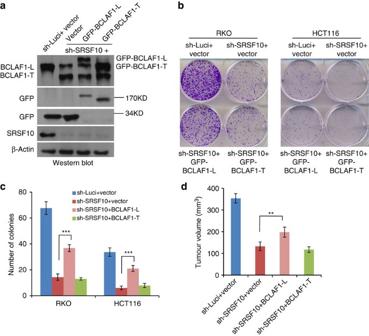Figure 7: BCLAF1-L rescues the biological effects of shSRSF10 cells. (a) RKO/shSRSF10 or RKO/shLuci cells were transfected with GFP-BCLAF1-L, GFP-BCLAF1-T or control vector, and selected for neomyocin resistance. Overexpression of GFP-BCLAF1-L or GFP-BCLAF1-T was confirmed by western blotting using indicated antibodies. (b) Clonogenic survival assay of RKO cells or HCT116 cells as described ina. (c) Quantization of the number of colonies for the indicated cell lines. Three independent experiments were performed and error bars indicate s.d. of mean. (d) Four indicated RKO cells as described inawere injected into nude mice, and tumour volumes were measured at the end of 35 days and represented as average size of tumour (mm3). Error bars indicate s.d. of mean. Full size image Figure 7: BCLAF1-L rescues the biological effects of shSRSF10 cells. ( a ) RKO/shSRSF10 or RKO/shLuci cells were transfected with GFP-BCLAF1-L, GFP-BCLAF1-T or control vector, and selected for neomyocin resistance. Overexpression of GFP-BCLAF1-L or GFP-BCLAF1-T was confirmed by western blotting using indicated antibodies. ( b ) Clonogenic survival assay of RKO cells or HCT116 cells as described in a . ( c ) Quantization of the number of colonies for the indicated cell lines. Three independent experiments were performed and error bars indicate s.d. of mean. ( d ) Four indicated RKO cells as described in a were injected into nude mice, and tumour volumes were measured at the end of 35 days and represented as average size of tumour (mm 3 ). Error bars indicate s.d. of mean. Full size image Increased SRSF10 parallels BCLAF1-L levels in CRC samples We next asked whether expression of SRSF10 is upregulated in clinical CRC samples. To this end, we examined its expression levels in the above 100 pairs of human CRC samples and their matched normal colorectal tissues by real-time RT–PCR ( Fig. 8a ). Expression levels were shown as a ratio between SRSF10 and the reference gene β-actin to correct for the variation in the amounts of RNA. Upregulation of SRSF10 (>2-fold) occurred in 32 of 100 (32%) CRCs compared with the paired normal colorectal tissues. Univariate analysis showed that mRNA levels of SRSF10 was significantly different between paired normal and cancer samples ( P <0.0001). In addition, the increased expression of SRSF10 could be associated with higher tumour grade ( P =0.0036; Supplementary Table 2 ). Significantly, a positive correlation was observed between SRSF10 expression levels and dysregulated ratio of BCLAF1 splice variants (5a+/5a−) in clinical samples ( Fig. 8b ). Similar correlation was also observed at protein levels between SRSF10 and BCLAF1-L in both cancer cell lines and clinical samples ( Supplementary Fig. 9 ). Together, these results indicate that SRSF10 is involved in CRC development, probably reflecting its ability to regulate alterative splicing of BCLAF1 pre-mRNA. 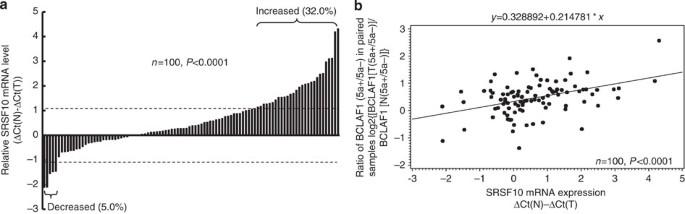Figure 8: Increased SRSF10 parallels BCLAF1-L levels in CRC samples. (a) Relative expression ofSRSF10mRNA in paired human CRC and normal tissues. Real-time PCR was performed on 100 paired CRC RNA samples. Expression levels ofSRSF10were normalized to that ofβ-actin. Data were calculated from triplicates. Bar value is the log ratio ofSRSF10expression levels between CRC (T) and matched normal tissues (N) from the same patient. Bar value ≤1 representsSRSF10is decreased in tumours. Bar value >1 represents thatSRSF10is increased in tumours. (b) Positive correlation betweenBCLAF15a+/5a− ratio and expression levels ofSRSF10was observed in CRC samples. Relationships between these two variables were determined by Pearson’s correlation coefficients. The correlation was analysed using SAS software. Figure 8: Increased SRSF10 parallels BCLAF1-L levels in CRC samples. ( a ) Relative expression of SRSF10 mRNA in paired human CRC and normal tissues. Real-time PCR was performed on 100 paired CRC RNA samples. Expression levels of SRSF10 were normalized to that of β-actin . Data were calculated from triplicates. Bar value is the log ratio of SRSF10 expression levels between CRC (T) and matched normal tissues (N) from the same patient. Bar value ≤1 represents SRSF10 is decreased in tumours. Bar value >1 represents that SRSF10 is increased in tumours. ( b ) Positive correlation between BCLAF1 5a+/5a− ratio and expression levels of SRSF10 was observed in CRC samples. Relationships between these two variables were determined by Pearson’s correlation coefficients. The correlation was analysed using SAS software. Full size image In this study, our data showed that SRSF10 activates inclusion of BCLAF1 exon5a to generate BCLAF1-L protein isoform. Both SRSF10 and BCLAF1-L stimulate cell proliferation and colony formation in vitro and promote tumorigenic capacity of colon cancer cells in mice. Importantly, elevated SRSF10 mRNA levels and increased inclusion rate of BCLAF1 exon5a observed in clinical CRC samples not only have a significantly positive correlation between them, but also correlated with the tumour grade of the patients. Thus, it is reasonable to propose that SRSF10 regulates tumorigenesis of colon cancer cells through alternative splicing regulation of BCLAF1 pre-mRNA and aberrant alterative splicing is a major contributor to cancer development. We here provided strong evidence that SRSF10 directly regulates alternative splicing of BCLAF1 pre-mRNA. Our previous experiments dealing with SRSF10 indicated that the protein functions as a sequence-specific activator, both in in vitro and in vivo assays, and can regulate alternative splicing of the GluR-B and cardiac triadin pre-mRNA [19] , [20] . The proposed mechanism for SRSF10 activation involves the stabilization of the binding of U1 and U2 snRNPs to the 5′-splice site and branch site, respectively [19] . Therefore, when binding within the alternative exon, SRSF10 could activate exon inclusion, which was further collaborated by transcriptome analysis of SRSF10-regulated splicing events in chicken cells [21] . The RNA binding in vitro and in vivo , in vivo splicing analysis with BCLAF1 pre-mRNA and RNA-seq analysis provided strong evidence to demonstrate that BCLAF1 is indeed a direct SRSF10 target. Misregulated alterative splicing events are very commonly observed and are involved in CRC development/progression [15] , [32] . For example, alterations in alterative splicing of the APC , K-Ras and TP53 genes have been implicated in the context of multiple carcinogenesis of CRC [15] . In addition, upregulation of typical SR proteins such as SRSF1 and SRSF6 was previously observed in colon cancers, although misregulated splicing events by them have not been identified [33] , [34] . These findings suggested that genetic lesions or dysregulation of splicing factors that affect alternative splicing are likely to contribute significantly to the aetiology of disease. In this study, knockdown of SRSF10 and BCLAF1-L demonstrated that these proteins play an essential role in colon cancer growth. More importantly, our data showed that SRSF10 regulation of BCLAF1 pre-mRNA splicing is a critical pathway in tumorigenesis of colon cancer cells. Beyond the involvement of BCLAF1 pre-mRNA, other SRSF10-regulated splicing targets could also implicate in this process, as more dramatic cancer-related phenotypes were observed by SRSF10 knockdown than BCLAF1-L knockdown. With RNA-seq analysis for identification of other splicing targets, future studies will be required to investigate roles of those splice isoforms in cancer development. Meanwhile, it will also be of interest to determine how the regulatory splicing networks involving the SR proteins, including SRSF10, functions in the carcinogenesis of CRC. We also provided multiple lines of evidence to demonstrate a pro-tumorigenic role for BCLAF1-L in colon cancer cells. Both knockdown and overexpression of BCLAF1-L, SSO treatment against BCLAF1 pre-mRNA and introduction of the L isoform into SRSF10 knockdown cells, all support this conclusion. It seems unlikely that BCLAF1-L acts as an apoptosis inducer as originally reported for the protein. Rather, the protein functions as an important modulator for cell adhesion and cell proliferation in cancer cells, as BCLAF1-L was highly expressed in colon cancer cells compared with normal epithelial cells ( Supplementary Fig. 9a ) and no significant effects was observed on colony formation of BCLAF1-L knockdown in normal epithelial cells ( Supplementary Fig. 10 ). Given the diverse roles observed for BCLAF1 in a variety of seemingly unrelated processes, this probably reflects cell context-dependent functions by BCLAF1. However, the molecular basis for its multiple functions remains to be defined. BCLAF1 was originally reported to associate with Bcl2 family members and acted as a transcriptional repressor [1] ; however, domain prediction does not reveal any structural similarities between BCLAF1 and these proteins. The most striking feature of BCLAF1 was RS-rich region (Arg-Ser repeats) that was observed at the amino terminal [2] . RS domain is typical of splicing factors that are involved in pre-mRNA biogenesis and pre-mRNA splicing [8] , [10] . Consistent with this, findings from several groups indeed indicate a role of BCLAF1 in pre-mRNA splicing [4] , [35] . As phosphorylated RS domain of splicing factors is well known to mediate multiple protein–protein interactions [8] , it is possible that different protein interactions involving BCLAF1 might induce distinct functions at different cellular contexts. Fully in line with this hypothesis, mass-spectrometry studies identified more than 30 phosphorylation sites within BCLAF1 (ref. 36 ). In addition, GSK3 was also predicted to directly phosphorylate BCLAF1, as treatment with the GSK3 inhibitor lithium results in a 3.7-fold decrease of phosphorylation of BCLAF1 at S531 (ref. 37 ). Further elucidation of protein factors interacted with BCLAF1-L will probably provide valuable insights into its mechanistic pathway in cancer cell growth. In summary, our findings reveal tumorigenic roles for SRSF10 and BCLAF1 L isoform in colon cancer cell growth and CRC development. We also identify SRSF10 as a key splicing regulator in controlling BCLAF1 pre-mRNA splicing and that SRSF10 regulation of BCLAF1 pre-mRNA splicing plays an important role in mediating tumorigenesis of colon cancer cells. Cell culture and reagents Human colon cancer RKO cells and human embryonic kidney 293T cells were cultured in DMEM medium, and HCT116 and HT29 cells were cultured in McCoy’s 5A, supplemented with 10% fetal bovine serum, 100 U ml −1 penicillin and 100 μg ml −1 streptomycin. All cells were incubated at 37 °C in a humidified atmosphere containing 5% CO 2 . α-Tubulin and β-actin antibodies were from Santa Cruz Biotechnology (Santa Cruz, CA). BCLAF1 and SRSF2 antibodies were from Merck Millipore (Billerica, MA). SRSF1 antibody was from Invitrogen (Camarillo, CA). Ki-67 antibody was from BD Biosciences (Bedford, MA). HA tag was from Abcam (Cambridge, MA). SRSF10 antibody was from Manley’s lab as previously described [38] . In addition, the growth-factor-reduced Matrigel was from BD Biosciences. Human CRC samples One hundred pairs of primary CRC and their corresponding adjacent normal tissues were obtained from CRC patients treated at Zhongshan Hospital (Shanghai, China) after their written informed consent. The fresh samples were snap-frozen in liquid nitrogen and stored at −80 °C until analysis. RT–PCR, western blotting, gel-shift assays and in vivo CLIP RNA extraction and reverse transcription were all carried out as described previously [39] . Briefly, total RNAs were extracted from indicated cell lines and reverse transcription was performed using oligo (dT) priming and M-MLV Reverse Transcriptase according to the manufacturer’s instructions (Promega Corporation, Madison, WI). For PCR analysis, primers were listed in Supplementary Table 3 . Quantification of all gene transcripts was carried out by real-time PCR using the SYBR Premix Ex Taq kit (TaKaRa, Otsu, Shiga, Japan). β-Actin was used as internal control. Western blotting and gel-shift assays were carried out as previously described [20] , [39] . Briefly, for western blotting, equal amounts of whole cellular extracts were subjected to 10% SDS–PAGE gels and detected using indicated antibodies. Uncropped images of western blots are shown in Supplementary Fig. 11 . For gel-shift assay, SRSF10 protein and in vitro transcribed radiolabelled BCLAF1 RNA probes were incubated under the splicing conditions. Products were analysed by 5% non-denaturing PAGE and autoradiography. In vivo CLIP (crossliking followed by immunoprecipitation) of BCLAF1 exon5a mRNA bound to SRSF10, SRSF1 and SRSF2 proteins was performed as previously described, with slight modifications [40] . Each of HA-tagged pcDNA3.0-SRSFs or empty vector controls was transiently transfected into 293T cells, and ultraviolet cross-linking was performed at 400 mJ cm −2 with a Stratalinker ultraviolet cross-linker (Stratagene). Immunoprecipitation was done with anti-HA antibody (Abcam ab9110, 5 μg per reaction) [41] -coupled protein A/G magnetic beads (50 μl per reaction) by using Magna RIP kit (Millipore). RNA was extracted from the immunoprecipitate and cDNA was synthesized with random primers. RNA enrichment was measured by RT–PCR with primers specific for BCLAF1-L exon5a1, 5a2 and 5a3. Details of primer sequences were provided in Supplementary Table 3 . siRNA, generation of viruses and stable cell lines Different siRNA oligos were ordered from Gene Pharma (Shanghai, China), and their respective sequences were listed in Supplementary Table 3 . The cells were transfected with siRNA oligos using LipofectamineRNAiMAX (Invitrogen, Carlsbad, CA). Ad-shSRSF10 adenovirus and control Ad-shLacZ adenovirus were generated in 293A cells as previously described [42] , [43] . Briefly, DNA fragments encoding shRNAs against SRSF10 or LacZ (as the negative control) were introduced into pENTR/U6 vectors and then recombinant vectors were propagated in 293A cells to produce adenoviruses. sh-SRSF10 retrovirus and sh-BCLAF1-L retrovirus were generated with pSiREN-puro retroviral vectors in 293 GPG cells as previously described [44] . RKO and HCT116 cells were infected with retroviruses either expressing Luci-shRNA, SRSF10-shRNA, or BCLAF1-L1- and 2-shRNA, respectively. Medium was replaced 24 h after infection, and after another 24 h incubation infected cells were selected by the addition of puromycin (2 μg ml −1 ) for 72–96 h. The GFP-Btf plasmid containing BCLAF1-L cDNA has also been described previously [45] . Transfection was performed using Lipofectamine reagent with a 1:2 DNA/Lipofectamine ratio, according to the manufacturer’s instructions. Cell proliferation and colony-survival assay Cell proliferation was measured by counting the number of the cells. Briefly, triplicate plates of cells were trypsinized and stained with Trypan blue, and unstained cells were counted using a haemocytometer. Colony-survival assay was performed as previously described [46] . Briefly, cells were seeded sparsely (2,000 cells per well for 6-well plates, 1,000 cells per well for 12-well plates) and were grown for 10 days with normal medium. Colonies were fixed and stained with 0.5% crystal violet solution in 20% methanol. Pictures of the plates were taken using Canon G9 digital camera and the number of colonies formed under each condition was scored from six random areas for each group. Xenograft tumour formation in mice Xenograft tumour formation assay was conducted as previously described [47] . In brief, 4-week-old male nude mice (BALB/cA-nu/nu) were obtained from Shanghai Experimental Animal Research Center and maintained in pathogen-free conditions. The mice were subcutaneously injected with indicated cells (3 × 10 6 cells in 100 μl serum-free media containing 0.25v/v matrigel) at each flank. All animals were maintained and used in accordance with the guidelines of the Institutional Animal Care and Use Committee of the Institute of Nutritional Sciences. Finally, mice were killed and tumours were extracted for further analysis. Immunostaining Xenografts harvested from three mice of each treatment group were formalin-fixed and paraffin-embedded as described previously [42] . Briefly, excised tumours from indicated groups were fixed in 4% buffered formalin for 16 h, and processed by the conventional paraffin-embedded method. To determine the apoptotic cells in tumours, the paraffin-embedded tumour sections (5 μm thick) were stained with the TUNEL kit (Promega Corporation) following the manufacturer’s instruction. The nucleus of the cells was stained with propidium iodide. Ki-67 staining was performed as previously described. Briefly, antigen retrieval was done by incubating the sections in 10 mM citrate buffer (pH 6.0) in a microwave for 10 min, followed by the incubation with 5% block serum for 1 h. Sections were then incubated with Ki67 antibody (1:100) at 4 °C overnight. Sections were examined microscopically and representative field were photographed under × 40 magnifications. RNA-Seq and data analysis Total RNAs isolated from RKO cells transfected with siSRSF10 or control siRNA were subjected to paired-end RNA-Seq using Illumina HiSeq 2000 system according to the manufacturer’s instruction. Reads mapping and data analysis for differentially regulated exons between two samples were carried out as previously described [21] . In brief, reads were mapped to a reference human genome and transcriptome using TopHat. Data analysis was carried out according to ASD software [21] , to detect the differentially regulated exons between the two samples. To identify the significantly changed alternative splicing events, a Fisher’s exact test was performed for each event using a 2 × 2 contingency table consisting of the read counts from either the inclusion or exclusion isoforms in the two samples.The raw sequence data and processed data have been submitted to Gene Expression Omnibus with accession number GSE 57325 . Microarray experiment and data analyses Total RNA was extracted from RKO stable cell lines expressing sh-Luci or sh-BCLAF1-L1. Gene expression was measured using a whole human genome microarray (Human Genome U133 Plus 2.0, Affymetrix Inc., Santa Clara, CA). A two-class unpaired method in the Significant Analysis of Microarray software (SAM, version 3.02) was applied to identify significantly differentially expressed genes between the two groups. Genes were determined to be significantly differentially expressed using fold change of 1.5 and q -value <5% as cutoffs in the SAM output result. Further functional analyses for biological processes were performed by using MAS (CapitalBio Molecule Annotation System) with differential expressed genes on the array. The level of significance was set at a P -value of 0.05 by Fisher’s exact test. Statistical analysis All data presented as histograms refer to a mean value±s.d. of the total number of independent experiments. Statistical analysis was performed by Student’s t -test at a significance level of P <0.05. Quantification of western blottings and RT–PCR was done by using ImageJ software, version 1.43u. For clinical CRC samples, statistical analyses were performed using the SAS software (version 8.2, SAS Institute Inc., Cary, NC). How to cite this article: Zhou, X. et al . BCLAF1 and its splicing regulator SRSF10 regulate the tumorigenic potential of colon cancer cells. Nat. Commun. 5:4581 doi: 10.1038/ncomms5581 (2014). Accession codes: Gene expression profiling data have been deposited in GEO under accession number GSE52990 .